Growth of high-density horizontally aligned SWNT arrays using Trojan catalysts Single-walled carbon nanotube (SWNT)-based electronics have been regarded as one of the most promising candidate technologies to replace or supplement silicon-based electronics in the future. These applications require high-density horizontally aligned SWNT arrays. During the past decade, significant efforts have been directed towards growth of high-density SWNT arrays. However, obtaining SWNT arrays with suitable density and quality still remains a big challenge. Herein, we develop a rational approach to grow SWNT arrays with ultra-high density using Trojan catalysts. The density can be as high as 130 SWNTs μm −1 . Field-effect transistors fabricated with our SWNT arrays exhibit a record drive current density of −467.09 μA μm −1 and an on-conductance of 233.55 μS μm −1 . Radio frequency transistors fabricated on these samples exhibit high intrinsic f T and f MAX of 6.94 and 14.01 GHz, respectively. These results confirm our high-density SWNT arrays are strong candidates for applications in electronics. In the past 20 years, marked advances in single-walled carbon nanotube (SWNT)-based integrated circuits (ICs) have been witnessed [1] , [2] . However, the density and quality of SWNT arrays still limit the performance of devices. In 2013, the scientists of IBM projected that, the desired density of SWNT arrays should be higher than 125 SWNTs μm −1 to realize the SWNT-based IC applications [3] . Several methods have been developed to produce high-density SWNT arrays, including post-treatment approaches and in situ growth methods [4] , [5] , [6] , [7] , [8] , [9] , [10] , [11] , [12] . In the case of post-treatment approaches, the multiple transfer method could obtain SWNT arrays with the density as high as 55 SWNTs μm −1 (ref. 5 ). However, these transferred SWNTs are not as aligned as as-grown SWNTs, which could lead to increased tube-to-tube interactions and degenerate the SWNTs’ quality. Meanwhile, Langmuir–Blodgett [6] and Langmuir–Schaefer [7] methods can also be utilized to increase the density of SWNT arrays, which can reach 500 SWNTs μm −1 . Nevertheless, post-treatment inevitably brought contamination, and the tubes were very short and in poor orientation, which cannot meet the requirement of high-performance devices. For the in situ growth methods, especially in chemical vapour deposition (CVD) systems, multiple loading catalyst [8] , multiple-cycle growth [9] , CuCl 2 /polyvinylpyrrolidone alcohol solution growth [4] and periodic growth [10] have been developed and the density can reach 10–50 SWNTs μm −1 . These SWNT arrays show good qualities and perfect alignment, but densities are still not high enough for SWNT-based IC applications [3] , [11] . To ensure SWNT quality and alignment, in situ growth of high-density SWNT arrays has many advantages. In the CVD process, the catalyst is a key factor for growing SWNTs on substrates [12] , [13] , [14] . How to maintain the activity of catalysts [15] , [16] , give catalyst nanoparticles more opportunities to nucleate SWNTs [9] , [17] and provide new catalysts during SWNT growth [8] are key issues for obtaining SWNT arrays with ultra-high density on substrates. In this study, ultra-high density of SWNT arrays were realized through use of Trojan catalysts. 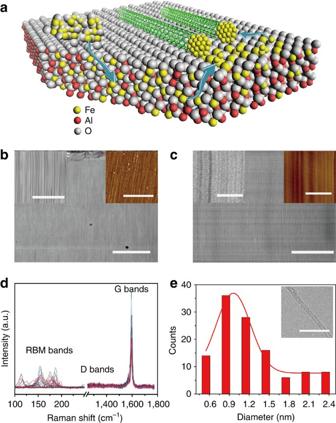Figure 1: Schematic illustration of growth mechanism and characterization of high-density SWNT arrays. (a) Schematic illustration of growing high-density horizontally aligned single-walled carbon nanotube arrays using Trojan catalysts. (b,c) SEM and AFM images of the as-grown SWNT arrays on sapphire surface at low and high magnifications, respectively, (insets: left SEM images, right AFM images). AFM and SEM images (insets inc) at higher magnification confirm that the density of SWNT arrays is as high as 130 SWNTs μm−1. (d) Raman spectra of the as-grown SWNT with 514.5 nm excitation. (e) Diameter distribution of the as-grown SWNT arrays (insets: HRTEM image of an individual SWNT). The red solid lines are Gaussian fitting peaks. Scale bar, 50 μm (b) (scale bar, 3 μm for the insets inb). Scale bar, 300 nm (c) (scale bar, 50 nm for the insets inc). Scale bar, 10 nm (e). Figure 1a schematically illustrates the procedure of the approach. First, the catalyst’s precursor was loaded onto the substrate by spin coating. After a high-temperature annealing process, the catalysts dissolve into the substrate and then become stored. Catalysts can then be released gradually under hydrogen atmosphere during growing process. As the gradual release mode reduces the interaction between active catalysts, which could lead to the deactivation of catalysts [18] , [19] , [20] , [21] , our growth mode obviously increases the efficiency of catalysts, and realizes the ultra-high density of SWNT arrays. The substrate acts as a catalyst container and the catalysts hide in the container. We named these catalysts as Trojan catalysts by analogy with soldiers emerging from the Trojan horse in the Greek story. Figure 1: Schematic illustration of growth mechanism and characterization of high-density SWNT arrays. ( a ) Schematic illustration of growing high-density horizontally aligned single-walled carbon nanotube arrays using Trojan catalysts. ( b , c ) SEM and AFM images of the as-grown SWNT arrays on sapphire surface at low and high magnifications, respectively, (insets: left SEM images, right AFM images). AFM and SEM images (insets in c ) at higher magnification confirm that the density of SWNT arrays is as high as 130 SWNTs μm −1 . ( d ) Raman spectra of the as-grown SWNT with 514.5 nm excitation. ( e ) Diameter distribution of the as-grown SWNT arrays (insets: HRTEM image of an individual SWNT). The red solid lines are Gaussian fitting peaks. Scale bar, 50 μm ( b ) (scale bar, 3 μm for the insets in b ). Scale bar, 300 nm ( c ) (scale bar, 50 nm for the insets in c ). Scale bar, 10 nm ( e ). Full size image Characterization of high-density SWNT arrays From scanning electron microscope (SEM) observations ( Fig. 1b,c ), uniform ultra-high-density SWNT arrays with large area were obtained using Trojan catalysts. Figure 1c shows an area with 1 μ width. The average nanotube density is measured to be at least 130 tubes μm −1 based on the number of the black lines, which were taken as SWNTs in the SEM image [22] . Higher-magnification SEM and atomic force microscope (AFM) images (insets in Fig. 1c ) further clearly indicate the density of the as-grown horizontally aligned SWNT arrays is as high as 130 SWNTs μm −1 . This is the highest reported density of grown SWNT arrays to date. Raman spectra of the high-density SWNT arrays with 514.5 nm excitation ( Fig. 1d ) show a distribution of radial breathing mode peaks between 110 and 190 cm −1 and the barely noticeable D band at a high-frequency region, which indicate that the aligned SWNT arrays are of high quality. High-resolution transmission electron microscopy observations on the as-grown sample revealed that only SWNTs were found (inset in Fig. 1e ). We observe that arrays grown in this fashion always consist of individual SWNTs, which is consistent with those reported in literature [23] , [24] . Furthermore, AFM measurements ( Fig. 1e ) show the main diameter distribution of the SWNT arrays from 0.8 to 1.6 nm with an average diameter of 1.26 nm. The dissolve-and-release mechanism for Trojan catalysts To realize the growth of SWNT arrays with high density, one possibility is to change the loading method of catalyst precursors onto the substrate. Loading catalyst precursors over time has been proved to be useful in high-density growth [8] . The key point of these methods is that newly loaded catalysts can be active during the SWNT growth process, which increases the density of as-grown SWNT arrays. To further improve the density of catalysts, we first proposed the continuous formation of catalyst nanoparticles during SWNT growth through a novel catalyst design. We attempted to hide the catalyst precursor inside the substrate before the CVD growth process. Under proper conditions, the catalyst precursor should be able to release from the substrate to form catalyst nanoparticles over time. We noted that the structure of sapphire (α-Al 2 O 3 ) and haematite (α-Fe 2 O 3 ) are very similar, as well as the diameter of low-spin Fe 3+ and Al 3+ (more details are given in Supplementary Fig. 1 and Supplementary Table 1 ). This indicates that Al 3+ can be replaced partly by Fe 3+ in the sapphire substrate. By a simple thermodynamic analysis in Supplementary Fig. 2 , this process is driven by entropy, for the chaos of the system will increase during the inter-infiltration between the adjacent crystal surfaces, until the components of these two surfaces verge to the same. To verify our assumption, Fe(OH) 3 /ethanol solution was deposited on the surface of the sapphire substrate by spin coating. 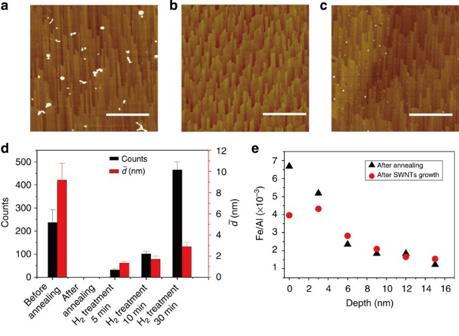Figure 2: Verification of the catalyst-dissolving and -releasing processes. (a) AFM images of substrate after spin-coating Fe(OH)3alcohol solution. (b) AFM images of sapphire substrate with loaded catalysts after annealing in a meffle furnace. (c) AFM images of substrate after H2treatment for 30 min. (d) The counts and average diameters of catalyst particles statistics in the areas (3μm × 3μm) after different treatment conditions: before and after annealing, H2treatment for 5, 10 and 30 min, respectively. The error bars of counts were s.d. that were calculated from five time statistic results. (e) XPS depth analysis of the substrates after annealing and after SWNTs growth. Scale bar, 1μm. Then the substrate was treated by 1,100 °C annealing for 8 h. Figure 2a and Fig. 2b show the AFM analysis of the surface morphology of sapphire before and after annealing process, respectively. The particles on the surface in Fig. 2a , which were known to be Fe(OH) 3 nanoparticles, were not found in Fig. 2b . To ensure that Fe(III) had dissolved into the bulk phase of sapphire instead of being volatilized during the annealing process, we performed depth profiling after removing the surface layer by argon bombardment, which is given in Fig. 2e . The content of Fe(III) had an exponential decrease with increasing depth in the substrate. To exclude the possibility that the sputtering itself causes the diffusion of the iron precursor, we loaded the catalyst precursor on sapphire by spin coating, as shown in Fig. 2a , and then performed X-ray photoelectron spectroscopy (XPS) depth profiling without any annealing process. The result is shown in Supplementary Fig. 3 . From what we can see, only the first plot shows a relatively high percentage of Fe. Fe signals are too weak to be observed in deeper sites. These results can be a strong evidence to provide strong evidence that Fe(III) has dissolved into the substrate. Figure 2: Verification of the catalyst-dissolving and -releasing processes. ( a ) AFM images of substrate after spin-coating Fe(OH) 3 alcohol solution. ( b ) AFM images of sapphire substrate with loaded catalysts after annealing in a meffle furnace. ( c ) AFM images of substrate after H 2 treatment for 30 min. ( d ) The counts and average diameters of catalyst particles statistics in the areas (3μm × 3μm) after different treatment conditions: before and after annealing, H 2 treatment for 5, 10 and 30 min, respectively. The error bars of counts were s.d. that were calculated from five time statistic results. ( e ) XPS depth analysis of the substrates after annealing and after SWNTs growth. Scale bar, 1μm. Full size image As we all know, Fe 2 O 3 can be reduced to Fe by H 2 treatment, but Al 2 O 3 cannot. Thus, dissolved Fe(III) could be reduced to Fe and form nanoparticles on the surface, which could act as catalysts to grow high-density SWNT arrays. To ensure that dissolved Fe(III) could afford the requirements of catalyst nanoparticles in high-density SWNT arrays, we deeply analysed the XPS data, as shown in Supplementary Fig. 4 . We found that only 1.54% of the Al 3+ was replaced by Fe 3+ in the first layer of sapphire. Meanwhile, Supplementary Fig. 5 showed that if 0.1% of the Fe(III) in the first layer was reduced to Fe and formed the nanoparticles, we can get a high-density horizontal SWNT array with 150 SWNTs μm −1 in density and 200 μ in length. Furthermore, Fe was not a unique case of the Trojan catalysts. Similar phenomena were observed in Fe, Mn and Co, but not found in Mo and Cu (more details are shown in Supplementary Fig. 6 and Supplementary Table 2 ). Most ions with similar diameters and same valence as Al 3 + can dissolve into sapphire, which could be regarded as an extension of the Trojan catalysts. Under our CVD growth condition at 830 °C, Fe 2 O 3 can be reduced to Fe in hydrogen ambience [25] . Fe 2 O 3 nanoparticles without any treatment can be reduced rapidly. In our Trojan catalysts, Fe(III) was dissolved into the substrate, which decreased the contact area between Fe(III) and H 2 . Thus, the reduction rate slows down intuitively. This ensures a continuous supply of Fe and realizes the gradual formation of the catalysts. Figure 2c shows the AFM analysis of the sapphire surface after a 30-min treatment with H 2 . Nanoparticles can be observed to be denser than those in Fig. 2b . Before the annealing process, the diameters of the particles were larger and the shapes of the particles were anomalous. After an annealing and reduction process, the nanoparticles became smaller and denser with a more regular geometrical shape, which was more suitable to act as catalysts. We also studied the relationship between reduction time and the topography of catalyst nanoparticles. Figure 2d shows the areal density (bars in black) and the diameter (bars in red) variation for the different treatment times with H 2 . We can see that with the additional reduction time, the diameter of the nanoparticle changed not obviously, while the areal density of the nanoparticles increases distinctly (more details are shown in Supplementary Fig. 7 ). The phenomenon could be a good proof that when Fe (III) are dissolved into the sapphire substrate, the reduction rate slows down obviously. Furthermore, the dissolve-and-release process also increases the density of catalysts and decreases the diameter of catalyst nanoparticles. To analyse the reduction process, especially the reaction site in the sapphire substrate, we performed another XPS depth analysis after the growth process, which is shown in Fig. 2e . We could see that the surface content of Fe (III) decreases significantly. This could be considered as the volatilization during H 2 treatment under high temperature during nanotube growth. The component of the substrate in a deeper area (>3 nm) remains, which means catalyst release, or Fe(III) reduction, mostly happened on the surface of the substrate (more details about XPS analysis are shown in Supplementary Fig. 8 ). These phenomena confirmed that H 2 treatment can release Fe from substrate gradually, which agreed with our catalyst design. To verify our hypothesis that the gradually released catalysts in the CVD process resulted in the increasing density of SWNTs, which is schematic illustrated in Fig. 3a , we performed three growth processes respectively on the same substrate under different CVD growth time. The sample was taken out from the furnace after the first growth of 5 min. After SEM characterization and annealing at 1,100 °C in air for 8 h, the same sample was put back into the furnace for the second growth under the same CVD conditions for 10 min. A third growth was performed the same as the second one, except the growth time was 30 min instead of 10 min. We compared the growth results in the same region with the help of marks on the sapphire substrate after every growth process. SEM images ( Fig. 3b–d ) showed the density of SWNT arrays gradually increased from <1 SWNTs μm −1 after the first growth to about 10 SWNTs μm −1 after the second growth and then reached the highest value (130 SWNTs μm −1 ) after the third growth. The density of SWNTs increased with the growth time extension, which means that new active catalysts formed continuously and catalysed the growth of new SWNTs. Furthermore, we attempted to grow SWNTs with other kinds of metals, such as Co and Mn, which were members of Trojan catalysts. As shown in Supplementary Fig. 9 , the density of the SWNT arrays can be increased with an annealing process after loading the catalyst than that without annealing. Differences among each metal in the density of arrays came from differences in the catalytic efficiency. This proved the universality of our Trojan catalysts. In addition, we utilized ion implantation technology to let the catalyst enter into the substrate [26] and successfully obtained high-density-aligned SWNT arrays as well ( Supplementary Fig. 10 ). This also confirmed the dissolving and releasing processes of Trojan catalysts. Thus, we believe that the gradually released catalysts are significant to obtaining ultra-high-density SWNT arrays. 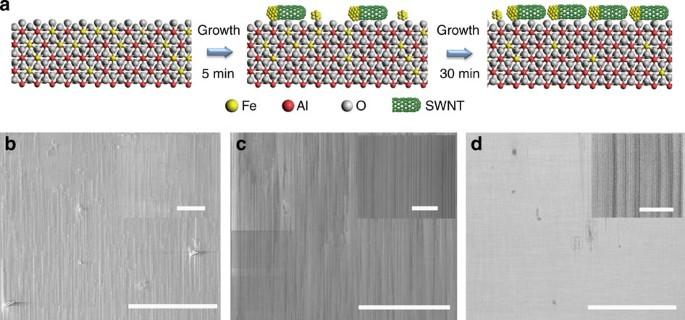Figure 3: The density of SWNTs increases with the growth time extension. (a) Schematic illustration of catalysts gradually released and catalysed the constant growth of SWNTs in the CVD process. (b–d) SEM images of SWNTs grown from the same catalyst area (marked with FFB) after the first CVD growth at 5 min (b), after the second CVD growth at 10 min (c) and after the third CVD growth at 30 min (insets: high-magnification SEM images). Scale bar, 100 μm (b–d) (inset inbis 20 μm, inset incis 1 μm and inset indis 200 nm). Figure 3: The density of SWNTs increases with the growth time extension. ( a ) Schematic illustration of catalysts gradually released and catalysed the constant growth of SWNTs in the CVD process. ( b – d ) SEM images of SWNTs grown from the same catalyst area (marked with FFB) after the first CVD growth at 5 min ( b ), after the second CVD growth at 10 min ( c ) and after the third CVD growth at 30 min (insets: high-magnification SEM images). Scale bar, 100 μm ( b – d ) (inset in b is 20 μm, inset in c is 1 μm and inset in d is 200 nm). Full size image Electrical properties of high-density SWNT arrays Experimental and theoretical works have demonstrated that the dense-aligned SWNT arrays are important and desirable for the applications of nanotube-based electronics, such as ICs and radio frequency (RF) electronics [27] , [28] . To evaluate the electrical performance of such ultra-high-density-aligned SWNT arrays, top-gated field effect transistors (FET) based on our as-grown SWNT arrays were fabricated directly on the growth substrate, and the electrical transport measurements were carried out in both d.c. and a.c. domains. 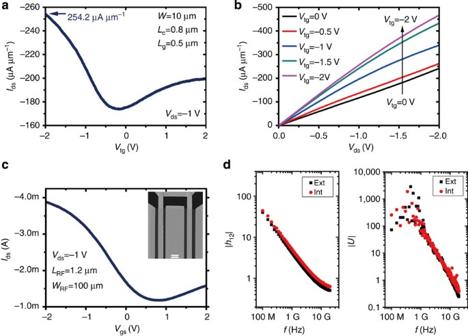Figure 4: High performance of high -density SWNT arrays devices. (a) Transfer characteristics of a high-current density device.Vds=−1 V. (b) Output characteristics of the high-current density devices.Vtgvaries from 0 to −2.0 V in steps of 0.5 V.W=10 μm,Lch=0.8 μm,Lg=0.5 μm. (c) Transfer characteristics of the RF transistor. Inset: SEM of the RF transistor. Scale bar, 2 μm.WRF=2 × 50 μm,LRF=1.2 μm andVds=−1 V. (d) The extrinsic (black dots) and intrinsic (red dots) current gain |h21| and power gain |U| as a function of frequency. Figure 4a,b present the d.c. electrical characterization of the fabricated FETs, where the channel length L ch is 0.8 μm, gate length L g is 0.5 μm, and channel width W is 10 μm. It is seen that the largest on-state current could even reach −467.09 μA μm −1 at V ds = V gs =−2 V, corresponding to an on-conductance of 233.55 μS μm −1 . As we know, the current density, or on-conductance, is the best results ever reported based SWNT arrays at the same scale of our channel length, and even match the results of solution-based SWNT arrays with a nanotube density of more than 500 tubes per μm, although the channel length of our device is almost 10 times larger [7] , [29] . This remarkably high current density and transconductance derives from the high density and perfect quality of our as-grown SWNT arrays. To further demonstrate the superiority of our high-density and quality SWNT arrays, we also measured the high-frequency performance of the fabricated RF transistors with L g2 =1.2 μm and W 2 =100 μm. Transfer characteristics of RF FETs are presented in Fig. 4c , where the SEM of the device structure was displayed as an inset. As shown in Fig. 4d , the extrinsic cutoff frequency f T and maximum oscillation frequency f MAX achieved are 5.13 and 11.33 GHz, respectively, which are comparable to the best performance of SWNT array-based RF transistors [28] . The intrinsic f T and f MAX of our RF transistor are 6.94 and 14.01 GHz, respectively, after the de-embedding process. As f T is associated with short-circuit current gain and f MAX reflects the unilateral power gain, the latter is a much more important and practical figure of merit in analogue circuit application. The highest intrinsic f MAX of an SWNT array-based transistor is about 30 GHz, where the channel length is about 100 nm. Therefore, our 1.2-μm-length transistors with an intrinsic f MAX of 14.01 GHz reveals a great potential for application of in situ grown SWNT arrays in the future RF electronics. Figure 4: High performance of high -density SWNT arrays devices. ( a ) Transfer characteristics of a high-current density device. V ds =−1 V. ( b ) Output characteristics of the high-current density devices. V tg varies from 0 to −2.0 V in steps of 0.5 V. W =10 μm, L ch =0.8 μm, L g =0.5 μm. ( c ) Transfer characteristics of the RF transistor. Inset: SEM of the RF transistor. Scale bar, 2 μm. W RF =2 × 50 μm, L RF =1.2 μm and V ds =−1 V. ( d ) The extrinsic (black dots) and intrinsic (red dots) current gain | h 21 | and power gain | U | as a function of frequency. Full size image In summary, a facile and effective strategy for growing high-density SWNT arrays was developed. We could obtain ultra-high-density (>130 SWNTs μm −1 ) horizontally aligned SWNT arrays through the use of Trojan catalysts, which is the highest density of grown SWNTs ever reported. Systematic experiments were performed to verify the catalyst-dissolving and -releasing processes by AFM, XPS, SEM and ion implantation technology. In addition, RF circuits based on the Trojan catalyst-synthesized nanotubes could have great potential for SWNT applications in future nanoelectronics. Trojan catalysts are useful for understanding the mechanism of SWNTs growth as well. Furthermore, combining s-SWNT arrays growth with Trojan catalysts, desired s-SWNT arrays with high density will be achieved. Furthermore, Trojan catalysts provide a new strategy for SWNT growth, but are not limited to SWNT growth. The essence of our Trojan catalysts is to release catalysts gradually and further to increase the efficiency, which is not limited to any kind of particular category of catalysts nor the growth of SWNT arrays with high density. It should be taken as a universal method and should be applicable for the catalyst-assisted fabrication of other one-dimensional nanomaterials, such as Si, Ge, GaN and ZnO nanowires or nanotubes and so on. Synthesis of high-density-aligned SWNT arrays In particular, a-plane sapphire substrates (single-side polished, miscut angle <0.5°, surface roughness <5 Å) were purchased from Hefei Kejing Materials Technology Co., China. After cleaning, the sapphire substrates must undergo a necessary annealing process (at 1,100 °C in air for 8 h) for better crystallization (see Supplementary Fig. 11 ). A total of 0.05 mmol l −1 Fe(OH) 3 /ethanol solution, which was used as a catalyst precursor, was dispersed onto the sapphire substrates by the spin-coating method. Then, the sapphire substrates with iron species on the surface were followed by a second annealing process (at 1,100 °C in air for 8 h as the same as stated above) for the iron species to dissolve into the sapphire substrates. The SWNT growth was performed in a furnace with a 1-inch tube. The sapphire substrates with well-dispersed iron species were put into the tube and heated in air to the desired temperature. After the system was purged with 300 standard cubic centimeters per minute (s.c.c.m.) argon, a flow of hydrogen (100 s.c.c.m.) and argon (50 s.c.c.m., through an ethanol bubbler) were introduced for ultra-high-density growth SWNT arrays at 830 °C for 30 min. Combining with ion implantation technology The clean a-plane sapphire substrates were annealed at 1,100 °C in air for 8 h in advance, then were implanted at room temperature with a mass-analysed beam of Fe ions (15 keV) to fluences of 1 × 10 15 to 1 × 10 16 Fe cm −2 . After ion implantation, the substrate undergoes another annealing process (at 1,100 °C in air for 8 h) for eliminating the surface defects. Subsequently, the growth process of SWNT arrays followed the same procedure as mentioned above. Characterization of high-density SWNT arrays The as-grown SWNTs were inspected with SEM (Hitachi S4800 field emission, Japan), AFM (Veeco NanoScope IIIA, Veeco Co.) and a Raman spectrometer (Horiba HR800 Raman system) to characterize the morphology, structure and electrical transport properties. XPS (ESCALab250, Thermo Scientific Corporation) and AFM were used to confirm the chemical composition and morphology of the substrate surface. Fabrication and measurements of electrical devices Devices were fabricated through a self-aligned U-gate process [30] , [31] . A bilayer e-beam resist with continuously varying sensitivity was used for defining the U-shaped top-gate stack, after electron-beam lithography and develop, 12 nm HfO 2 and 70 nm Ti were sequentially deposited by atomic layer deposition and electron-beam evaporation followed with a traditional lift-off process. The pad of the source, drain and gate was composed of Ti/Pd/Au 0.5/30/50 nm, and the channel was defined through reactive ion etching using oxygen plasma. Ten nanometres of Pd was finally deposited as a self-aligned contact layer. The d.c. characteristics of our devices were measured in a vacuum cryogenic probe station (Lakeshore TTP4) with a semiconductor analyzer (Keithley 4200 SCS). The a.c. responses of our FETs were characterized by S-parameter measurements and it was carried out on a microwave probe station with GSG probes (Cascade 9000) in atmosphere. The de-embedding process was based on a short-open-load-through scheme. How to cite this article: Hu, Y. et al . Growth of high-density horizontally aligned SWNT arrays using Trojan catalysts. Nat. Commun. 6:6099 doi: 10.1038/ncomms7099 (2015).